π–π interaction of aromatic groups in amphiphilic molecules directing for single-crystalline mesostructured zeolite nanosheets One of the challenges in material science has been to prepare macro- or mesoporous zeolite. Although examples of their synthesis exist, there is a need for a facile yet versatile approach to such hierarchical structures. Here we report a concept for designing a single quaternary ammonium head amphiphilic template with strong ordered self-assembling ability through π–π stacking in hydrophobic side, which stabilizes the mesostructure to form single-crystalline mesostructured zeolite nanosheets. The concept is demonstrated for the formation of a new type of MFI (zeolite framework code by International Zeolite Association) nanosheets joined with a 90° rotational boundary, which results in a mesoporous zeolite with highly specific surface area even after calcination. Low binding energies for this self-assembling system are supported by a theoretical analysis. A geometrical matching between the arrangement of aromatic groups and the zeolitic framework is speculated for the formation of single-crystalline MFI nanosheets. The development of macro- or mesoporous zeolitic materials with hierarchical pore architectures is of increasing importance for researchers in porous materials science, because the sole presence of micropores in bulk zeolites can cause diffusion limitations and limit their widespread use as industrial catalysts [1] , [2] , [3] , [4] . There are several methods to prepare hierarchical zeolites such as top-down desilication by alkali post-synthetic modification [5] , bottom-up directed assembly by self-assembly of various zeolite seeds [6] and by templates. Much attention has been focused on the synthesis of zeolites with desired pore structure using soft and hard templates, such as surfactants [7] , [8] , [9] , cationic polymer [10] , polystyrene beads [11] , mesoporous silica [12] and carbon materials [13] , [14] , [15] . Although much considerable progress has been made in developing strategies to direct the formation of porous zeolites, designing a templating strategy for obtaining ordered hierarchical pore structures with crystallographically ordered zeolite remains an unsolved challenge. Quaternary ammonium species are well known as zeolite templates because of their strong interactions with the inorganic framework [16] , [17] , [18] , [19] . Long-chain alkyl–quaternary ammonium molecules are universally used to synthesize mesoporous silica materials through the self-assembled liquid crystal templating route [20] , [21] , [22] . Recently, Ryoo and coworkers [8] succeeded in synthesizing polycrystalline mesostructured MFI (zeolite framework code by International Zeolite Association) zeolite using designed bifunctional surfactants [7] , [8] , [23] , in which the connection of the head groups of the multiple quaternary ammoniums to hydrophobic alkyl chains is the indispensable factor for the effective structure-directing agent to simultaneously form MFI zeolite and a mesoscale micellar structure. However, directing the structure of zeolite using longer alkyl chain lengths and simple one-head quaternary molecules is generally an energetically unfavourable event compared with the use of multiple quaternary ammonium head groups [8] , [20] , [24] . The high synthetic energy in one-head quaternary groups would disrupt the formation of their lamellar structure. An approach to designing feasible templates for the synthesis of hierarchical zeolites is to stabilize the micelle structure by introducing highly rigid segments that have strong interactions with each other in the hydrophobic chain to block crystal growth by forming an extremely stable hydrophobic layer and that form an ordered orientation to provide a geometric match with the MFI zeolitic framework. Aromatic–aromatic or π–π stacking interactions are well known as effective noncovalent intermolecular forces, which are normally employed for H-type or J-type stacking of aromatic groups with ring centroid–centroid distances of ~\n3.3–3.8 Å [25] , [26] , [27] . In particular, they can facilitate self-assembly or molecular recognition processes while involving extended structures that are constructed from building blocks with aromatic moieties to matching MFI nanosheet [28] , [29] . The presence of at least two benzene rings is known to be necessary for the formation of stable bilayer assemblies of amphiphiles [30] . Therefore, energetically stable micellar structures and their ordered orientation would make the single-head amphiphilic template for directing the formation of mesostructured zeolite nanosheets possible. In this study, first, we introduce biphenyl and naphthyl into the alkyl tail of an amphiphilic template with a single quaternary ammonium head group to form C 6 H 5 –C 6 H 4 –O–C 10 H 20 –N + (CH 3 ) 2 –C 6 H 13 (Br − ) (denoted as C Ph–Ph-10-6 ) and C 6 H 4 –C 4 H 3 –O–C 10 H 20 –N + (CH 3 ) 2 –C 6 H 13 (Br − ) (C Nh-10-6 ) (see Supplementary Figs 1–4 ), which give rise to single-crystalline mesostructured zeolite nanosheets with a lamellar structure (SCZN-1). Second, MFI nanosheets joining with a 90° rotational boundary (SCZN-2) are templated using bolaform amphiphilic molecules with bi-quaternary ammonium head groups and biphenyl groups C 6 H 13 –N + (CH 3 ) 2 –C 6 H 12 –N + (CH 3 ) 2 –(CH 2 ) n –O–C 6 H 4 –C 6 H 4 –O–(CH 2 ) n –N + (CH 3 ) 2 –C 6 H 12 –N + (CH 3 ) 2 –C 6 H 13 (4Br − ) (BC Ph-n-6-6 , Supplementary Figs 5–10 ). 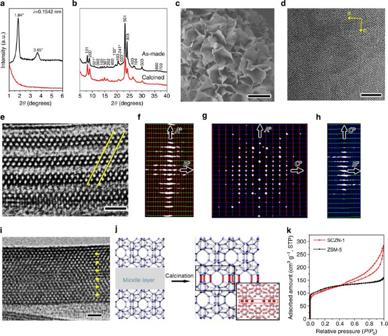Figure 1: Structural characterization of SCZN-1 templated by CPh–Ph-10-6 Low- (a) and high-angle (b) XRD patterns of the as-made SCZN indicating the highly ordered lamellar structure. The peaks of the calcined material in the low-angle XRD pattern disappeared due to the removal of the template. (c) SEM image revealing that the as-made sample possessed a petal-like morphology. (d,e) high-resolution transmission electron microscopy (HRTEM) image taken along the [010] and [100] axis of the as-made SCZN. (f–h) 3D EDT projections with multiple unit cell meshes along different directions illustrating the structural details in 3D reciprocal space. (i) HRTEM image taken along the [100] axis of the calcined sample that reveals the formation of MFI single crystal. (j) Structural model of SCZN before and after calcination. (k) The N2adsorption–desorption isotherms of calcined SCZN-1 and conventional ZSM-5. The synthesis molar composition was 1 CPh–Ph-10-6: 20 SiO2: 2.5 Na2O: 0.2 Al2O3: 800 H2O. The scale bars inc,d,eandirepresent 2 μm, 20 nm, 5 nm and 5 nm, respectively. Synthesis and characterization of SCZN-1 Figure 1a shows the low-angle X-ray diffraction (XRD) pattern (transmission mode) of the as-made sample synthesized with C Ph–Ph-10-6 as a template. Two well-resolved peaks at 2θ=1.84° and 3.65° were indexed as the first- and second-order reflections of layered MFI nanosheets with new unit cell constant B =4.8 nm ( A and C are same as MFI unit), indicating a periodic interlamellar structural order. The electron charge distribution curve ( Supplementary Fig. 11 , Supplementary Note 1 ) revealed different scattering powers between the MFI and micelle layers. The thickness of the MFI layer was estimated to be ~\n2.7 nm, corresponding to the observation from TEM (vide post). Most of the sharp peaks in the high-angle range ( Fig. 1b ) were associated with the h 0 l reflections of the MFI framework, suggesting good crystallinity in the a–c plane. However, the limited information and considerable peak overlapping caused difficulties in distinguishing between the h 0 l and 0 kl reflections in the powder XRD pattern and determining the super mesostructure. Figure 1: Structural characterization of SCZN-1 templated by C Ph–Ph-10-6 Low- ( a ) and high-angle ( b ) XRD patterns of the as-made SCZN indicating the highly ordered lamellar structure. The peaks of the calcined material in the low-angle XRD pattern disappeared due to the removal of the template. ( c ) SEM image revealing that the as-made sample possessed a petal-like morphology. ( d , e ) high-resolution transmission electron microscopy (HRTEM) image taken along the [010] and [100] axis of the as-made SCZN. ( f – h ) 3D EDT projections with multiple unit cell meshes along different directions illustrating the structural details in 3D reciprocal space. ( i ) HRTEM image taken along the [100] axis of the calcined sample that reveals the formation of MFI single crystal. ( j ) Structural model of SCZN before and after calcination. ( k ) The N 2 adsorption–desorption isotherms of calcined SCZN-1 and conventional ZSM-5. The synthesis molar composition was 1 C Ph–Ph-10-6 : 20 SiO 2 : 2.5 Na 2 O: 0.2 Al 2 O 3 : 800 H 2 O. The scale bars in c , d , e and i represent 2 μm, 20 nm, 5 nm and 5 nm, respectively. Full size image The scanning electron microscopy (SEM) images ( Fig. 1c and Supplementary Fig. 12 ) revealed that the sample was composed of uniform flower-like morphology with a petal thickness of ~\n30 nm. Recently developed three-dimensional electron diffraction tomography (three-dimensional (3D) EDT) data provided single crystal information not only on the atomic structure of the nanosheets but also on the relative positions of successive sheets. Strong and sharp diffractions from the h 0 l plane revealed the high structural coherence of the MFI sheets. The super lattice resulting from registered MFI layers was determined to be rhombic with cell parameters of A =20.5 Å, B =40.3 Å and C =13.9 Å. The spatial correlation of layers along the b axis was indicated by spots along the b * axis, the diffusion of which might come from the existence of amphiphilic molecules as well as deviation from the superstructure. The single-crystalline mesostructure could be directly observed in high-resolution transmission electron microscopy images ( Fig. 1d,e ), where MFI layers were organized along the B direction to form a super mesostructure. In particular, crystallographically ordered MFI layers could connect with each other to MFI single crystals by forming new Si-O-Si bonds after calcination ( Fig. 1i,j ), with maintaining morphology. Therefore, it can be concluded that SCZN has been synthesized by C Ph–Ph-10-6 (we denoted it as SCZN-1). The N 2 desorption–desorption isotherms of calcined SCZN-1 shows a similar profile with conventional bulk MFI zeolite due to the similar single-crystalline structure with conventional ZSM-5. It shows the uptake steps below P/P 0 =0.02 due to micropore filling or capillary condensation ( Fig. 1k and Supplementary Fig. S4 ), which is present in all conventional zeolite samples, as compared with ZSM-5 (ref. 31) [31] . The hysteresis loop of SCZN-1 at a relative pressure range of 0.5–1.0 shows a few amount and random distribution of mesopores due to the interconnected single-crystalline pore system and some polycrystalline pores formed by random aggregation of the thin petals. The Brunauer–Emmett–Teller (BET) surface area, micro- and mesopore volumes of SCZN-1 were measured to be 395 m 2 g −1 , 0.12 cm 3 g −1 and 0.30 cm 3 g −1 , respectively, similar to those of conventional ZSM-5 ( Supplementary Fig. 13 ). The relatively low BET surface area also confirmed the formation of a MFI single crystal after calcination, while polycrystalline MFI zeolite with a high surface area was obtained after calcination due to the large amount exposure of ac plane as reported by Ryoo [8] . Similarly, the template C Nh-10-6 can also produce SCZN-1 ( Supplementary Fig. 14 ). Our strategy was also successfully extended to the bolaform amphiphilic molecules with the single quaternary ammonium head ( Supplementary Fig. 15 ). Synthesis and characterization of SCZN-2 It is well known that rotational boundaries are commonly found in MFI zeolite with an overgrown relationship between the ( h 00) and (0 k 0) faces [32] , [33] , which increases the possibility of the construction of a hierarchical structure with a large surface area and pore volume. The approximate cell parameters of a and b in MFI and the similar 10-ring pores provide a fundamental possibility for the occurrence of the phenomena of intergrowth on itself, which is inherent to the MFI structure. Several small molecules [34] , [35] , [36] , in particular, the dimers of the tetrapropyl ammonium bromide cation can generate structural constraints or stresses and can easily form the boundaries of MFI crystals. However, the mesoscopic porosity in these materials cannot be controlled with small structural-directing agents (SDAs) alone, which always resulted in the mesoporous structure with broad pore size distributions. Here, we rationally designed a series of bolaform amphiphilic molecules with bi-quaternary ammonium head groups and biphenyl groups (BC Ph-n-6-6 ), which could act as particular cationic dimers, to direct a new type of hierarchical SCZN with uniform mesopore size due to the presence of their hydrophobic parts (we denoted these samples as SCZN-2). 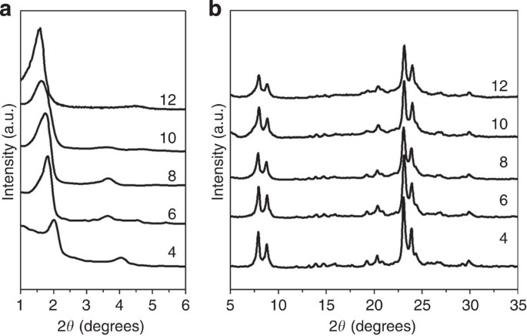Figure 2: XRD PAtterns. Low- (a) and high-angle (b) XRD patterns of as-made samples. They are synthesized by bolaform templates with different hydrophobic carbon chain, BCPh-n-6-6(n=4, 6, 8, 10, 12), all indicating the construction of SCZNs. The initial gel composition was 1 BCPh-n-6-6: 20 SiO2: 2.5 Na2O: 0.2 Al2O3: 800 H2O. Figure 2 shows the XRD patterns of the as-made SCZNs synthesized with BC Ph-n-6-6 ( n =4, 6, 8, 10, 12). All samples show ordered lamellar structures. The first-order reflections were gradually shifted to a smaller 2 θ value as the carbon chain increased from 4 to 12 with a distinct interlamellar spacing ( d (1) ) of 4.37 nm (2 θ =2.02°, n =4), 4.83 nm (2 θ =1.83°, n =6), 4.93 nm (2 θ =1.79°, n =8), 5.29 nm (2 θ =1.67°, n =10) and 5.52 nm (2 θ =1.60°, n =12). The high-angle XRD patterns reveal the crystal structure of layered MFI, which includes only the h 0 l reflections. As shown in Fig. 3 , the SEM images revealed that all of these SCZNs have an extraordinary boundary structure with the 90° rotation of adjacent faces. However, it was found that the number of 90° rotational crystals appears at a significant level and dominant house-of-cards-like morphologies were observed only in the samples templated by BC Ph-6-6-6 and BC Ph-8-6-6 , compared with the other three samples. The others synthesized by BC Ph-n-6-6 ( n =4, 10, 12) show only limited amounts of intergrowth without house-of-cards-like structure. This result suggests that only proper chain lengths (for example n =6 and 8 of BC Ph-n-6-6 ) are favourable for the formation of house-of-cards-like joining with 90° rotational crystals. Figure 2: XRD PAtterns. Low- ( a ) and high-angle ( b ) XRD patterns of as-made samples. They are synthesized by bolaform templates with different hydrophobic carbon chain, BC Ph-n-6-6 ( n =4, 6, 8, 10, 12), all indicating the construction of SCZNs. The initial gel composition was 1 BC Ph-n-6-6 : 20 SiO 2 : 2.5 Na 2 O: 0.2 Al 2 O 3 : 800 H 2 O. 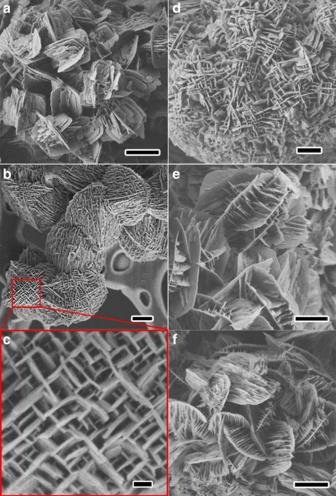Figure 3: SEM images of as-made samples shown inFig. 2. BCPh-4-6-6(a), BCPh-6-6-6(b,c), BCPh-8-6-6(d), BCPh-10-6-6(e), BCPh-12-6-6(f), all showing the formation of SCZNs with 90° rotational boundary. The scale bars ina,b,c,d,e,frepresent 1 μm, 500 nm, 100 nm, 500 nm, 1 μm and 1 μm, respectively. Full size image Figure 3: SEM images of as-made samples shown in Fig. 2 . BC Ph-4-6-6 ( a ), BC Ph-6-6-6 ( b , c ), BC Ph-8-6-6 ( d ), BC Ph-10-6-6 ( e ), BC Ph-12-6-6 ( f ), all showing the formation of SCZNs with 90° rotational boundary. The scale bars in a , b , c , d , e , f represent 1 μm, 500 nm, 100 nm, 500 nm, 1 μm and 1 μm, respectively. Full size image To analyse the internal boundary structure, the TEM images of thin sections of the as-made samples were observed. Taking the sample templated by BC Ph-6-6-6 as an example ( Fig. 4a,b ; Supplementary Fig. 16 ), the perpendicular crystal plates with a boundary relationship shared a common c axis, in which the (100) faces are overgrown on the (010) faces; a schematic representation of a structural model of the boundary is illustrated clearly in Supplementary Fig. 17 . Two independent layers join through chemical bonding on the ac plane and zig-zag channels of one layer are interconnected with straight channels of the other layer. The connectivity at the joints could arise through the formation of a new set of Si-O-Si bonds ( Supplementary Fig. 18 ), which would sustain the lamellar structure and improve its stability. From some ultrathin crossed nanosheets as shown in Fig. 3c (although not so many), it can be found that they penetrate into each other. Therefore, the connection with MFI/MEL twins is also possible in these intergrowth domains, which is the similar to Tsapatsis's report [34] . After the template molecule was removed by calcination in air, the MFI layers in the main plates collapsed to form single crystals, whereas the majority of the boundary layers did not completely collapse to produce clear mesopores because of the framework connectivity ( Fig. 4c,d ; Supplementary Fig. 19 ). In addition, the readily apparent house-of-cards-like morphology could construct a new macroporous system (~\n100 nm) due to the mutual pillaring between ultrathin plates ( Supplementary Fig. 20 ). Therefore, this type of SCZN-2 possesses well-defined micro–meso–macroporous architecture, even after calcination. 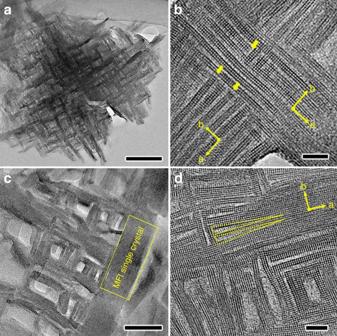Figure 4: High-resolution transmission electron microscopy (HRTEM) images of as-made and calcined SCZN-2 templated by BCPh-6-6-6. (a,b) TEM image taken along the commoncaxis of a slice of the as-made SCZN embedded in epoxy resin clearly revealing the 90° rotational boundary. (c,d) HRTEM images of the calcined sample demonstrating the presence of mesopores, even after calcination, because of the 90° rotational boundary. The scale bars ina,b,c,drepresent 200 nm, 10 nm, 50 nm and 10 nm, respectively. Figure 4: High-resolution transmission electron microscopy (HRTEM) images of as-made and calcined SCZN-2 templated by BC Ph-6-6-6 . ( a , b ) TEM image taken along the common c axis of a slice of the as-made SCZN embedded in epoxy resin clearly revealing the 90° rotational boundary. ( c , d ) HRTEM images of the calcined sample demonstrating the presence of mesopores, even after calcination, because of the 90° rotational boundary. The scale bars in a , b , c , d represent 200 nm, 10 nm, 50 nm and 10 nm, respectively. Full size image The representative TEM images ( Supplementary Fig. 21 ) of the other samples by BC Ph-n-6-6 show different degrees of intergrowth, once more confirming that only the templates with proper chain lengths are favourable for the formation of 90° rotational crystals. The cause of this result can be explained in terms of the geometric matching between the intergrowth crystal structure and the hydrophobic chain length of the bolaform templates. Based on the inherent characters of the MFI intergrowth structure (crystallographically correlative connectivity and uniform thickness of each MFI sheet, Supplementary Figs 17,18 ), three kinds of possible models with the narrowest space distance (corresponding to the molecular size used here) for the connectivity can be considered, exhibiting different distances ~\n4.0, 4.9 and 5.9 nm ( Supplementary Fig. 22 ). The as-made samples templated by BC Ph-n-6-6 all exhibit lamellar structure with the same MFI layer thickness of ~\n2.7 nm and interlamellar distance range from 4.37 to 5.52 nm, as confirmed from XRD patterns ( Fig. 2a ) and TEM observations ( Supplementary Fig. 23 ). The interlamellar spacing by BC Ph-6-6-6 and BC Ph-8-6-6 are found to be 4.83 and 4.93 nm, respectively, very close to 4.9 nm, while that by BC Ph-4-6-6 , BC Ph-10-6-6 and BC Ph-12-6-6 are 4.37, 5.29 and 5.52 nm, respectively, far away from the three model sizes. Therefore, it is reasonable to be considered that a high degree of matching between the molecular size and space distance between two adjacent MFI sheets would encourage successive rotational intergrowth. The XRD patterns ( Supplementary Fig. 24 ) of the calcined samples show that a broad Bragg peak existed in the samples templated by BC Ph-6-6-6 and BC Ph-8-6-6 , indicating the presence of abundant mesopores. 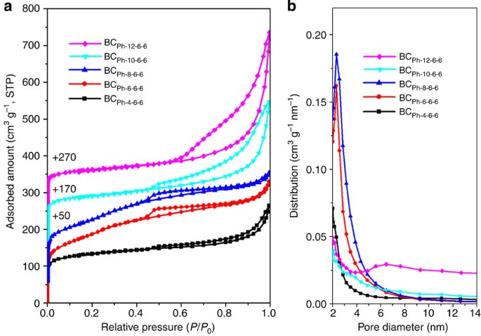Figure 5: Pore properties of calcined SCZN-2. The N2adsorption–desorption isotherms (a) and pore size distributions (b) of calcined SCZNs by BCPh-n-6-6indicating that abundant mesopores were retained only in the samples synthesized by BCPh-6-6-6and BCPh-8-6-6owning to the well 90° rotational boundary. Figure 5 shows the N 2 desorption–desorption isotherms of calcined samples by BC Ph-n-6-6 . All samples show the uptake steps below P/P 0 =0.02 due to the microporous MFI structure [31] , while only the samples templated by BC Ph-6-6-6 and BC Ph-8-6-6 exhibit a higher uptake at a relative pressure range of 0.2–0.8 due to the presence of abundant and uniform mesopores after calcination. The capillary condensation loop at P/P 0 =0.1–0.3 reveals the presence of small mesopores formed by the collapse of the lamellar structure near the joints ( Fig. 4d ), and the hysteresis loop at P/P 0 =0.5–0.7 indicates the presence of interconnected pores formed by the aggregation of card-like sheets. The BET surface area, micro-, and mesopore volumes of SCZN-2 were 658 m 2 g −1 , 0.11 and 0.51 cm 3 g −1 , respectively. The sharp peaks at 2.4 nm (approximately equal to the scale of one lamellar micelle) were clearly caused by the 90° rotational boundary relationship. However, the other three samples prepared from BC Ph-n-6-6 ( n =4, 10, 12) exhibited no obvious uptake at a relative pressure range of 0.2–0.8, no peaks in the pore size distribution curve and low BET surface areas ( Supplementary Table 1 ) owing to the presence of a reduced boundary structure, indicating the little amount of mesopores in these samples as has been shown in their SEM and TEM images. Figure 5: Pore properties of calcined SCZN-2. The N 2 adsorption–desorption isotherms ( a ) and pore size distributions ( b ) of calcined SCZNs by BC Ph-n-6-6 indicating that abundant mesopores were retained only in the samples synthesized by BC Ph-6-6-6 and BC Ph-8-6-6 owning to the well 90° rotational boundary. Full size image In addition, it was found that the intergrowth structure produced by BC Ph-6-6-6 was formed as the result of an in situ phase transformation process, specifically from amorphous to crystalline; this observation varies significantly from previous reports, that is, where a solution-mediated seed crystal growth mechanism was indicated in the small SDAs system [37] . As shown in the supporting information, the amorphous solid ( Supplementary Figs 25,26a ) then gradually yielded intermittent lattice fringes ( Supplementary Fig. 26b,c ), which were wide along the a axis and c axis; this observation provided sufficient evidence to justify the initial nucleation of MFI nanosheets and the structural units for subsequent 90° rotational growth. Along with further crystallization growth, SCZN with sufficient 90° rotational boundaries was gradually constructed ( Supplementary Fig. 26d,e ). The intergrowth crystals that reside perpendicular to each other grow through the process of in situ transformation, which involves an amorphous-to-crystalline evolution (or solid-state transformation mechanism). During this process, the crystals almost retained their initial size. As mentioned above, compared with the spontaneous crystallization growth of zeolitic nanosheets by small SDAs [33] , [34] , our strategy and the obtained products based on the self-assembly of amphiphilic molecules demonstrated the difference resulting from as well as the advantage of available control on uniform mesoscopic porosity, crystallographic correlation between two perpendicular crystals depending on the molecular size, the in situ transformation mechanism and structural stability. Theoretical study of amphiphilic molecules-directing SCZN First, to understand why the single-head quaternary ammonium amphiphilic molecules containing aromatic groups (C Ph–Ph-10-6 ) could form lamellar-structured MFI nanosheets, we applied molecular mechanics calculations to compare the relative stabilities of bulk and layered MFI zeolite structures with different template molecules: C Ph–Ph-10-6 , single-head C 22 H 45 N + (CH 3 ) 2 C 6 H 13 (C 22-6 ) and bi-head quaternary ammonium-type template C 22 H 45 N + (CH 3 ) 2 C 6 H 12 N + (CH 3 ) 2 C 6 H 13 (C 22-6-6 ) [8] . These computations were based on an assumption that both the bulk and layered zeolite structures could be formed at the initial stage of the synthesis, and the relative stability determines which form survives. Although a thorough study must be based on free energy comparisons, which are much more demanding and beyond the scope of this work, quick calculations based on energy minimization could provide the most essential information, despite they are only qualitatively correct. The calculations were based on energy minimizations using the Martini coarse-grained (CG) models for the amphiphilic molecules and atomic model for the zeolites [38] . These force fields have been tested for relevant molecules and applied in this work based on the common (Lorentz–Berthelot) combination rules. The bulk models were constructed using experimental XRD data. The layered models were represented by a slab model with 4 × 3 repeat units along the a and c directions, and the thickness of MFI layer ( b directions) were fixed using available experimental values. The surfaces of the layered models were saturated with OH groups. The 3D periodic boundary condition was applied. The interlayer space was filled with the side groups of SDAs and filled with water molecules so that the density is 1.0 g cm −3 . The average binding energies between the amphiphilic molecules and the zeolite frameworks were calculated to evaluate the stabilities. The relative stabilities were calculated by subtracting the binding energies of the bulk model from that of the nanosheet model. The results are summarized in Table 1 , and the details of the calculations are given in Supplementary Figs 27,28 , Supplementary Table 2 . Table 1 Calculated binding energies. Full size table The calculation result indicates that the bulk model (−104.5 kJ mol −1 ) is more stable than the layered one (−93.6 kJ mol −1 ) for C 22-6 , which is consistent with our experimental results. Using C 22-6 as the template, we obtained only bulk ZSM-5 crystals ( Supplementary Fig. 29 ), which is similar to those obtained using CTAB as SDA in the hydrothermal synthesis [39] ; we could not obtain MFI nanosheets by C 22-6 with numerous setting of the synthesis conditions. For C 22-6-6 , the layered structure (−114.0 kJ mol −1 ) is more stable than the bulk one (−152.2 kJ mol −1 ). As a matter of fact, Ryoo and co-workers have reported that the layered structures can be easily made by using C 22-6-6 as SDA. As the aromatic groups are introduced into the hydrophobic tail in C Ph–Ph-10-6 , our data shows that the layered structure (−439.6 kJ mol −1 ) is also more stable than the bulk one (−487.1 kJ mol −1 ). After combining the experimental data for the mesostructured MFI nanosheets synthesized by both C 22-6-6 and C Ph–Ph-10-6 , the calculation results indicate that the presence of both the second quaternary ammonium head and biphenyl groups in an amphiphilic molecule would significantly reduce the binding energies of the mesostructured zeolite synthesis system. Although both C Ph–Ph-10-6 and C 22-6-6 direct the formation of lamellar-structured nanosheets, close analysis of the calculated energies reveal that the stabilizations are due to quite different mechanisms. For C 22-6-6 , the electrostatic interactions between the quaternary ammonium groups outside of the slabs and the slab surfaces that otherwise do not exist in the bulk structure contribute the most to the binding energy. From the optimized configuration of C Ph–Ph-10-6 nanosheet model ( Supplementary Fig. 28 ), the distances between two phenyl rings are about 3 Å, indicating the π–π interactions among the biphenyl groups play an important role to stabilize the nanosheet model. In addition, the steric repulsions between the bulky aromatic groups and the MFI channels reduce the stability of the bulk structure. It is well known that the formation of a 90° rotational boundary always also entails high binding energies. However, the coexistence of bi-quaternary ammonium head and biphenyl groups would significantly reduce the total binding energies of mesostructured zeolite synthesis system. Therefore, from a theory angle, the bolaform amphiphilic molecules (BC Ph-n-6-6 ) could easily construct the intergrowth structure. The corresponding experimental results based on BC Ph-n-6-6 would strongly support the above calculations. Speculation of the arrangement manner of templates in SCZN To investigate the role of the template, the stereoregularity of C Ph–Ph-10-6 was studied using UV–visible absorption spectroscopy (Fig. 6a ). In a dilute water solution, C Ph–Ph-10-6 molecules were isolated from each other, resulting in absorption bands from the molecule itself at 199 nm (benzene ring) and 260 nm (biphenyl group). In the crystalline solid state, the packing of the template molecules was very close and regular and the interactions of biphenyl groups result in clear π–π stacking. The energy for the transition from the π highest occupied molecular orbital to the π* lowest unoccupied molecular orbital decreased due to π–π molecular orbital overlaps from the aromatic groups, which led to a red shift of the absorption bands of ~\n37 nm (at 297 nm). Identical absorption bands were also obtained from the as-made SCZN, which demonstrated the formation of similar π–π stacking interactions. 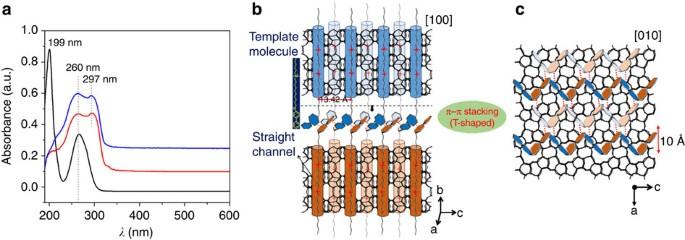Figure 6: Schematic representation of the formation of SCZN. (a) Ultraviolet–visible absorption spectra of template molecules (CPh–Ph-10-6) in a dilute water solution (the black line) showing absorption bands of the isolated molecule. A red shift to 297 nm in the crystalline solid (the red line) and in the as-made SCZN (the blue line) revealing the similar formation ofπ–πstacking between biphenyl groups due toπ–πmolecular orbital overlaps. (b) Single quaternary ammoniums in the template molecules are located in the straight channel and serve as a template to direct the formation of SCZN. (c) The arrangement of biphenyl groups from adjacent MFI layers along thea–cplane orientation matching the MFI frameworks. Figure 6: Schematic representation of the formation of SCZN. ( a ) Ultraviolet–visible absorption spectra of template molecules (C Ph–Ph-10-6 ) in a dilute water solution (the black line) showing absorption bands of the isolated molecule. A red shift to 297 nm in the crystalline solid (the red line) and in the as-made SCZN (the blue line) revealing the similar formation of π – π stacking between biphenyl groups due to π – π molecular orbital overlaps. ( b ) Single quaternary ammoniums in the template molecules are located in the straight channel and serve as a template to direct the formation of SCZN. ( c ) The arrangement of biphenyl groups from adjacent MFI layers along the a–c plane orientation matching the MFI frameworks. Full size image As mentioned above, the position of aromatic rings in the centre of micelles was confirmed by electron charge distributions based on the low-angle XRD data ( Supplementary Fig. 11 ). The intact configuration of C Ph–Ph-10-6 template without decomposition in SCZN was confirmed by 13 C nuclear magnetic resonance (NMR) spectra ( Supplementary Fig. 30 ). The thermogravimetric analysis combined with elemental analysis data (ratio of N/Si=0.035) indicate that not only that all micropores were directed by the quaternary ammonium groups, but also that one template corresponds to one micropore ( Supplementary Fig. 31 ). Therefore, it can be speculated that the single ammonium groups of the template molecules are located in the straight channel of the MFI framework to direct the formation of MFI micropores and the aromatic groups in the hydrophobic tails to form stable network with strong π–π stacking ( Fig. 6b ). From the top view of the biphenyl groups along the b direction, the arrangement of biphenyl groups from adjacent MFI layers along the a – c plane can also generate strong π–π stacking with the adjacent ones (red dotted lines, Fig. 6c , see Supplementary Figs 32,33 , Supplementary Note 2 for more detailed description). In this way, all of the biphenyl groups possess a favourable T-shaped configuration with a well-defined network, which geometrically matches the MFI frameworks and produce the crystallographically related single-crystalline MFI layers. This is also the reason why C 22-6-6 and C Ph–Ph-10-6 direct polycrystalline and single-crystalline MFI nanosheets, respectively. The arrangement of the biphenyl groups in BC Ph-6-6-6 was similar to that of C Ph–Ph-10-6 . ( Supplementary Figs 34–36 , Supplementary Note 3,4 ). However, such an arrangement remains speculative. Generally, the interaction distance and the stacking conformation of the aromatic rings can be effectively determined via X-ray crystallography. However, a suitable single crystal is required to obtain these data in conjunction with an X-ray single-crystal diffractometer. Unfortunately, the aromatic arrangement in the structures of our MFI nanosheets are limited to several layers ( Fig. 1e , Supplementary Fig. 12 ) and are separated by a layer-type zeolitic framework, which cannot be discerned using X-ray crystallography; therefore, the corresponding diffraction pattern cannot be detected. We aimed to design self-assembling, single-SCZN by introducing aromatic groups (such as biphenyl and naphthyl) into the hydrophobic tail of the amphiphilic molecule. The strong self-assembling ability and highly ordered orientation of aromatic groups through π–π stacking stabilize the lamellar micelle structure to make the amphiphilic molecules with single quaternary ammonium head group for directing SCZN possible. This was confirmed by single-crystal analysis with 3D EDT, powder XRD and EM. The low binding energies of this self-assembling system, obtained by computer simulation using molecular mechanics calculations, provided a theoretical evidence for the feasibility of our strategy. Furthermore, when the aromatic groups connected to the bolaform amphiphilic molecules in the hydrophobic region, a new type of hierarchical zeolite, in which the SCZN join with 90° rotational boundary, was obtained due to the special branch configuration of the bolaform molecule and the stronger π–π stacking around the boundary joints. Because of the chemically bonded connection at the crossed joints, the lamellar structures did not completely collapse, even after calcination, and they exhibited a highly specific surface area. The formation of SCZN with crystallographically correlated mesostructure from crystallized MFI units is probably the result of a geometrical match between aromatic groups and MFI zeolitic framework. We expect that our findings will provide new insight into the molecular factors governing the formation of the inorganic–organic mesophase and microporous materials, which would open up new possibilities for elaborately fabricating mesoporous zeolites. Synthesis of amphiphilic molecules C Ph–Ph-10-6 (1) The synthesis procedure was illustrated in Supplementary Fig. 1 . 4-phenylphenol (3.4 g, 20 mmol) and 1,10-dibromodecane (30 g, 100 mmol) were mixed in 250 ml of ethanol containing 1.2 g of KOH and refluxed under an N 2 atmosphere for 1 day. The product was filtered and washed repeatedly with C 2 H 5 OH several times to obtain the intermediate 9 . Then, 7.8 g (20 mmol) of 9 and 3.9 g (22 mmol) of N , N -dimethylhexylamine were mixed in 150 ml of acetonitrile and refluxed at 95 °C for 24 h. After cooling to room temperature, the product 1 was filtered, washed with diethyl ether, and dried in a vacuum oven overnight (9.6 g, 93%). The detailed characterization of these novel organic compounds was shown in Supplementary Methods . Synthesis of C Nh-10-6 (2) The synthesis of C Nh-10-6 followed the similar procedures for the preparation of 1 instead of the use of 2-naphthol. Synthesis of BC Ph-10-6 (3) 4,4′-biphenol (4.7 g, 25 mmol, TCI) and 1,10-dibromodecane (37.5 g, 125 mmol) were mixed in 300 ml of ethanol containing 3.0 g KOH and refluxed under an N 2 atmosphere. The product was filtered and washed repeatedly with hot C 2 H 5 OH and water to obtain 11 . Then, 11 (3.8 g, 10 mmol) and N , N -dimethylhexylamine (3.9 g, 22 mmol) were refluxed in 150 ml of acetonitrile. Solid product 3 was obtained after the crude product was filtered and washed with diethyl ether several times (8.3 g, 94%). Synthesis of BC Ph-n-6-6 (4–8) The detailed synthesis procedures were illustrated in Supplementary Fig. 5 . Take the preparation of BC Ph-10-6-6 ( 7 ) for an example, 12.5 g of 11 (20 mmol) and 43.0 g (0.25 mol) of N , N , N ′, N ′-tetramethyl-1,6-diaminohexane were mixed in 300 ml of acetonitrile/toluene (1:1) and stirred at 65 °C for 20 h. The intermediate 18 was filtered and washed with cold diethyl ether three times. The final product 7 was obtained by adding 4.8 g (5 mmol) of 18 and 4.2 g (25 mmol) of 1-bromohexane, followed by refluxing in 200 ml of acetonitrile for 1 days. After cooling to room temperature, the product was filtered, washed with diethyl ether and dried in a vacuum oven overnight (5.8 g, 90%). The amphiphilic molecules with different alkyl chain length (BC Ph-4-6-6 , BC Ph-6-6-6 , BC Ph-8-6-6 and BC Ph-12-6-6 ) were also obtained following the similar procedures. The intermediates 12 – 19 were synthesized through the similar methods for the preparation of 11 and 18 by substituting 1,10-dibromodecane with 1,4-dibromobutane, 1,6-dibromohexane, 1,8-dibromooctane and 1,12-dibromododecane, respectively, see Supplementary Methods for all of the characterization for these organic compounds. Synthesis of single-crystalline MFI nanosheets In a typical synthesis of MFI nanosheets, 0.518 g C Ph–Ph-10-6 template, 0.2 g NaOH, 0.0328, g sodium aluminate and 14.4 g distilled water were mixed together and stirred for ~\n0.5 h. Then, 4.16 g tetraethyl orthosilicate (98%) was added to yield a nominal molar composition of 1 C Ph–Ph-10-6 : 20 SiO 2 : 2.5 Na 2 O: 0.2 Al 2 O 3 : 800 H 2 O. The mixtures were stirred for an additional 2 h. Crystallization was conducted in Teflon-lined stainless steel autoclaves (25 ml) at 150 °C, with the autoclaves tumbling at 40 r.p.m. The products were filtered, washed with distilled water and dried at 100 °C overnight, and then they were calcined in air at 550 °C. The other zeolite materials were synthesized following similar procedures only with different templates. Characterization Powder XRD patterns were recorded on a Rigaku X-ray diffractometer D/max-IIIA equipped with a Cu Kα radiation source (40 kV, 30 mA) and transmission mode measurements were made on a PANalytical X’Pert with Cu Kα radiation (45 kV, 40 mA), fixed divergence slit of 1/4°, anti-scattering slit of 1/8°, a programme-controlled receiving slit (with constant irradiated length of 10 mm) and a step size of 0.0042° in transmission mode to reduce errors at small scattering angles in the Bragg–Bretano configuration. SEM was conducted on a JEOL JSM-7401F electron microscope operating at 1 kV. Zeolite thin section preparation was carried out after the mixing of epoxy resin and zeolite material with further solidifying. From the composite, thin sections with 50–60 nm thickness were prepared on a Leica EM UC7 Ultramicrotome with a diamond knife. The sections were then loaded on a TEM grid (400 mesh Cu). High-resolution transmission electron microscopy was performed using a JEOL JEM-3010 microscope operating at 300 kV ( C s=0.6 mm, resolution of 1.7 nm). Images were recorded with Kodak electron film SO-163 using low-electron dose conditions. 3D EDT data were collected on a JEOL JEM-2100 (LaB6 filament) with C s=1.4 mm operated at 200 kV. Herein, the total range of angles covered is 80° with 0.1° step. The nitrogen adsorption/desorption isotherms were measured at 77 K using an ASAP 2010 M+C analyser. The surface area was calculated by the BET method, and the pore size was obtained from the maxima of the pore size distribution curve calculated by the Barett–Joyner–Halenda method using the adsorption branch of the isotherm. Ultraviolet/visible diffuse reflectance spectra were recorded on a Perkin-Elmer Lambda 20 UV/Vis spectrometer, whereas the UV/Vis absorption spectrum of the filter was measured with a Shimadzu UV-2450 spectrophotometer. The absorbance spectra were obtained through a Kubelka–Munk transformation of the reflectance spectra. The element analysis of Si, Al and C, N was determined from the inductively coupled plasma analysis (ICP, Perkin-Elmer 3300DV) and Elementar Vario-ELIII IRMS analyser, respectively. Thermogravimetric analyses were performed on TGA 7 thermogravimetric analyser (Perkin-Elmer, USA). The heating rate was 20 °C min −1 . 1 H and 13 C NMR spectra were recorded on a Varian MERCURY plus-400 (400 MHz) spectrometer, and the chemical shifts are reported in p.p.m. relative to the residual deuterated solvent and the internal standard tetramethylsilane. The solid-state 13 C CP/MAS NMR spectra were collected on Oxford AS400 NMR spectrometer at 100 MHz using a sample spinning frequency of 3 kHz. HRMS for the organic compounds were performed on a Waters Micromass Q-TOF Premier Mass Spectrometer in positive model. Molecular mechanics calculations The relative stabilities of bulk and layer zeolite (MFI) structures due to different SDAs were investigated by using molecular mechanics calculations. SDAs were represented by the CG model, in which superatom types are defined for groups of atoms. A four-to-one mapping is used to represent the molecules in the simplified model; that is, on average, four atoms are represented by a single interaction centre. Different colours are used for different superatoms. C 1 , N 0 , SN and SC represent alkyl group, quaternary ammonium group, ethoxyl group and phenyl group. Three SDA molecules, denoted as C 22-6 , C 22-6-6 and C Ph–Ph-10-6 , were calculated, and the CG model is illustrated in Supplementary Fig. 27 . The red and yellow lines represent the MFI framework. Super water atoms are in deep blue. Except the species presented in Supplementary Fig. 27 , other species (salts, alcohols) that may be present in the synthesis were not considered. For MFI zeolite, the bulk (B) and layered (L) structures were considered. The bulk models were constructed using experimental XRD data. The layered models were represented by a slab model with 4 × 3 repeat units along the a and c directions, and the thickness of MFI layer (along the b directions) were fixed using available experimental values. For the layered structure C 22-6 -L for which there is no experimental data, the distance was determined according to the ratio of molecular lengths with respect to C 22-6 and C 22-6-6 . The cell-edge parameters for both bulk and layered structures are listed in Supplementary Table 2 . The surfaces of the layered models were saturated with OH groups. The 3D periodic boundary condition was applied. The initial configurations were set by placing the terminal quaternary ammonium groups (N0) in the centres of channel intersections of MFI. The two alkyl groups from one structure-directing agent (SDA) were placed in opposite orientations in the channel. The channel allows coexistence of two alkyl chains so that two alkyl chains from different SDAs are tangled in the channel. Therefore, one sees that two alkyl chains of C 22-6 or C 22-6-6 tangled in the channel, but one benzene ring of C Ph–Ph-10-6 in the channel. In the layered structures, parts of the SDA molecules are in the interlayers. Due to hydrophobic effect, water molecules are separated from the clusters of hydrocarbons. In addition, the interlayer space was filled with the side groups of SDAs and filled with water molecules so that the density is 1.0 g cm −3 . The configurations were optimized using the L-BFGS algorithm [40] with an energy tolerance of 10.0 kJ mol −1 nm −1 . A cutoff value of 1.0 nm was used for non-bond interactions. The calculations were conducted using GROMACS 4.5.5 (ref. 41) [41] . The optimized structures of the simulated models are shown in Supplementary Fig. 28 . The average binding energy ( E b ) between one SDA molecule and the MFI frameworks in either bulk or layered structure is defined as: where E [MFI+SDAs] is the total energy of MFI and SDAs, E [MFI] is the energy of MFI only and E [SDA] is the energy of SDA in isolation and n is the number of SDAs. The absolute binding energies between bulk and nanosheet zeolite structures are −104.5 kJ mol −1 and −93.6 kJ mol −1 for C 22-6 , −114.0 kJ mol −1 and −115.2 kJ mol −1 for C 22-6-6 , −439.6 kJ mol−1 and −487.1 kJ mol −1 for C Ph–Ph-10-6 , respectively. The absolute values for different template molecules cannot be directly compared, however, because different models are adopted for phenyl and alkyl groups, and the standard states do not correspond to synthesis solutions. How to cite this article : Xu, D. et al. π – π interaction of aromatic groups in amphiphilic molecules directing for single-crystalline mesostructured zeolite nanosheets. Nat. Commun. 5:4262 doi: 10.1038/ncomms5262 (2014).